Monitoring the dynamics of clonal tumour evolutionin vivousing secreted luciferases Tumours are heterogeneous cell populations that undergo clonal evolution during tumour progression, metastasis and response to therapy. Short hairpin RNAs (shRNAs) generate stable loss-of-function phenotypes and are versatile experimental tools to explore the contribution of individual genetic alterations to clonal evolution. In these experiments tumour cells carrying shRNAs are commonly tracked with fluorescent reporters. While this works well for cell culture studies and leukaemia mouse models, fluorescent reporters are poorly suited for animals with solid tumours—the most common tumour types in cancer patients. Here we develop a toolkit that uses secreted luciferases to track the fate of two different shRNA-expressing tumour cell clones competitively, both in vitro and in vivo . We demonstrate that secreted luciferase activities can be measured robustly in the blood stream of tumour-bearing mice to accurately quantify, in a minimally invasive manner, the dynamic evolution of two genetically distinct tumour subclones in preclinical mouse models of tumour development, metastasis and therapy. Tumours are heterogeneous cell populations composed of genetically distinct subclones. They arise through the reiterative process of clonal expansion, genetic diversification and selective outgrowth of clones that have a phenotypic advantage within a given microenvironmental context [1] , [2] , [3] , [4] , [5] , [6] . Fluctuations in clonal architecture can occur, for example, in the context of disease progression such as metastasis or drug treatment [4] , [7] . Therapeutic intervention may destroy cancer clones and erode their habitats, but it can also inadvertently provide a potent selective pressure for the expansion of resistant variants [3] . Importantly, genetic alterations that drive metastatic progression or relapse following cancer therapy are attractive targets for therapeutic intervention. However, given an average mutation frequency in tumours of more than one mutation per Mb [8] , [9] , pinpointing the individual genetic alterations that drive positive or negative selection in clonal evolution is far from trivial. Recently, reverse genetic engineering of loss-of-function phenotypes by RNAi technologies has provided a valuable tool to probe specifically the contribution of individual genes to cancer phenotypes in cell culture and animal models. Short hairpin RNAs (shRNAs) can be expressed from DNA-based vectors integrated into the genome and highly complex shRNA vector libraries can introduce experimental heterogeneity into previously clonal tumour cell lines that covers in principle the whole transcribed genome [10] , [11] . Clonal evolution of such experimentally engineered heterogeneous tumour cell populations in vitro and also in vivo has been profiled quantitatively by next generation sequencing of shRNAs that are positively or negatively selected over time [12] , [13] , [14] . Clonal analysis by sequencing of tumour DNA, however, is an endpoint assay and therefore provides only limited information about the dynamics of tumour evolution. To monitor clonal evolution in a time-resolved manner, shRNA expression has been coupled to fluorescent reporters, which can be tracked over time by fluorescence microscopy or flow cytometry. Changes in the percentage of fluorescent cells in the population inform about the disappearance or expansion of an shRNA-expressing subclone, respectively [15] . By adding a second fluorescent marker, a non-targeting shRNA can be monitored in parallel to control for non target-specific shRNA effects [16] . Fluorescent reporters have been used extensively to track different shRNA-bearing tumour cell populations competitively in cell cultures. In animals, this is limited to models where tumour cells are readily accessible for sampling and flow cytometry, for example, in the case of circulating leukaemia cells, since quantification of fluorescence by imaging techniques requires expensive instrumentation, is time consuming, involves frequent anaesthesia and is biased because of photon absorption as a function of wavelength, tissue and depth [13] , [17] , [18] . More than 90% of all tumours in cancer patients, however, are solid tumours. Representative samples from these tumours are not accessible in regular intervals for time course studies precluding the monitoring of their clonal architecture by direct analysis of tumour samples or fluorescence-based methods. In patients, it is routine clinical practice to monitor tumour growth using tumour-specific biomarkers detectable in the blood. Recently, the analysis of circulating tumour DNA in the plasma has been established as a novel genetic biomarker to monitor the evolution of distinct tumour subclones [19] . However, circulating tumour DNA is present in only low concentration and requires plasma sample volumes that cannot be obtained repeatedly from small animal models for time course studies [19] , [20] , [21] . We therefore predicted that artificial reporters secreted from the tumour cells into the circulation could serve as suitable surrogate markers. In this respect, a naturally secreted Gaussia princeps luciferase (GLuc) has been described as a highly sensitive reporter for localization of cells by bioluminescence imaging and for quantitative assessment of cells in vivo by measuring its concentration in blood [22] , [23] , [24] . Another naturally secreted Cypridina noctiluca luciferase (CLuc) [25] has similar properties but different substrate specificity allowing us to develop a dual-secreted luciferase assay for simultaneous monitoring of two differently labelled cell populations in a competitive culture setting. In this study, using lentiviral vectors for constitutive and doxycycline (dox)-regulated, luciferase-coupled expression of shRNAs we validate secreted luciferases for monitoring the clonal evolution of heterogeneous tumour cell populations during tumour progression, metastasis and therapy response both in cell culture and mouse models. Monitoring clonal evolution in cell culture To monitor clonal evolution of heterogeneous cell populations, we explored the use of secreted luciferases from GLuc and CLuc as bioluminescence markers. GLuc and CLuc have comparable emission spectra with peaks at λ max =480 nm and 465 nm, respectively [24] , [25] . We labelled HCT116 cells with GLuc or CLuc by lentiviral transduction ( Fig. 1a ). GLuc and CLuc activities in the cell culture supernatant were measured with high specificity and no detectable crosstalk using coelenterazine or vargulin as substrates, respectively, and correlated directly with cell number ( Fig. 1b,c ). GLuc and CLuc activities in the cell culture medium remained stable at −20 °C allowing for combined analysis of collected samples at the end of a time course experiment ( Supplementary Fig. 1 ). When GLuc + and CLuc + cells were mixed, the ratio of luciferase activities (G/C ratio) measured in the medium correlated with the mixing ratio of the cells and the cell ratio quantified independently by GLuc/CLuc-quantitative PCR (qPCR) at the level of genomic DNA isolated from the mixed cultures ( Fig. 1d , Supplementary Fig. 2 ). G/C ratios measured in the supernatant of long-term cultures remained constant over six orders of magnitude for more than 2 weeks of passaging indicating that expression of neither luciferase confers a selective disadvantage as a confounding source of experimental bias ( Fig. 1e ). As a model for monitoring clonal evolution in cell cultures, we labelled parental H460 cells with GLuc (H460 par ) and a cisplatin (CDDP)-resistant subclone with CLuc (H460 res ) by lentiviral transduction before mixing at a 1:1 ratio. G/C ratios in the culture medium remained constant in the vehicle control, but dropped by two orders of magnitude following CDDP treatment consistent with disappearance of GLuc + parental cells and overgrowth of the CDDP-resistant CLuc + subclone ( Fig. 1f ). 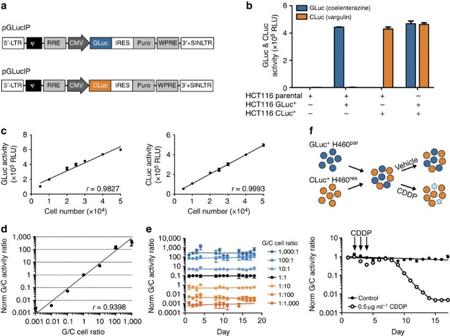Figure 1: Dynamic monitoring of clonal evolution in cell culture with secreted luciferases. (a) Lentiviral vectors for constitutive, puromycin-selectable cell labelling with GLuc and CLuc. (b) GLuc and CLuc activity measured in the supernatant of cultures containing parental, GLuc+and/or CLuc+HCT116 cells as indicated (n=3). (c) Correlation of GLuc and CLuc activity in the cell culture supernatant with cell number (n=3). (d) Correlation of GLuc/CLuc activity ratio (G/C ratio) in the cell culture supernatant with mixing ratio of GLuc+and CLuc+cells. G/C ratio was normalized to the 1:1 mixture (n=5). (e) Stability of the normalized G/C ratio in the supernatant of long-term cultures (n=3). (f) Parental cisplatin (CDDP)-sensitive (H460par) and resistant (H460res) H460 cell clones were labelled with either GLuc (GLuc+H460par) or CLuc (CLuc+H460res), mixed in a 1:1 ratio, cultured 3 days in the presence or absence of CDDP (arrows) and monitored daily for GLuc/CLuc activity in the culture supernatant (n=3). Shown is the G/C ratio normalized to day 1. All data are presented as mean±s.d. unless indicated otherwise. Correlation is indicated by the Pearson’s correlation coefficientr. Figure 1: Dynamic monitoring of clonal evolution in cell culture with secreted luciferases. ( a ) Lentiviral vectors for constitutive, puromycin-selectable cell labelling with GLuc and CLuc. ( b ) GLuc and CLuc activity measured in the supernatant of cultures containing parental, GLuc + and/or CLuc + HCT116 cells as indicated ( n =3). ( c ) Correlation of GLuc and CLuc activity in the cell culture supernatant with cell number ( n =3). ( d ) Correlation of GLuc/CLuc activity ratio (G/C ratio) in the cell culture supernatant with mixing ratio of GLuc + and CLuc + cells. G/C ratio was normalized to the 1:1 mixture ( n =5). ( e ) Stability of the normalized G/C ratio in the supernatant of long-term cultures ( n =3). ( f ) Parental cisplatin (CDDP)-sensitive (H460 par ) and resistant (H460 res ) H460 cell clones were labelled with either GLuc (GLuc + H460 par ) or CLuc (CLuc + H460 res ), mixed in a 1:1 ratio, cultured 3 days in the presence or absence of CDDP (arrows) and monitored daily for GLuc/CLuc activity in the culture supernatant ( n =3). Shown is the G/C ratio normalized to day 1. All data are presented as mean±s.d. unless indicated otherwise. Correlation is indicated by the Pearson’s correlation coefficient r . Full size image Monitoring clonal evolution in mice To explore the suitability of the two secreted luciferases for monitoring tumours in vivo , tumours were induced in mice by subcutaneous injection of HCT116 cells labelled with either GLuc or CLuc. Luciferase activities in blood samples of tumour-bearing mice yielded signals at least four orders of magnitude above background without detectable crosstalk ( Fig. 2a ). A single drop of ~10 μl blood was sufficient for reliable quantification of both luciferases. Ex vivo , there was negligible background activity and both luciferase activities were stable in whole blood and plasma samples for at least 1 h ( Supplementary Fig. 3 ). Luciferase activity in plasma samples was approximately 10-fold higher than in whole blood, likely because of light absorption by haemoglobin ( Supplementary Fig. 3 ). In vivo half-lifes of GLuc and CLuc were 10 and 90 min, respectively, suggesting only a minor contribution of luciferase accumulation over time to the total signal measured in blood samples ( Supplementary Fig. 4 ). GLuc + and CLuc + tumours were visualized independently with high sensitivity by bioluminescence imaging following sequential intravenous (i.v.) injection of the respective substrate ( Fig. 2b ). Subcutaneous injection of 1:1 mixtures of GLuc + and CLuc + HCT116 cells resulted in a parallel, exponential increase of both luciferase activities in the plasma that correlated well with tumour volume measured with calipers ( Fig. 2c ). However, while tumours became measurable after approximately 3 weeks, dual luciferase assays on plasma samples reliably detected tumour growth 1–2 weeks earlier. When mice were injected with different ratios of GLuc + and CLuc + cells, the luciferase ratio measured in the plasma of tumour-bearing mice directly correlated with the ratio of initially injected cells and the ratio measured by GLuc/CLuc-qPCR in the genomic DNA of explanted tumours ( Fig. 2d,e ). As a model for monitoring clonal tumour evolution in mice, GLuc + H460 par and CLuc + H460 res cells (see Fig. 1f ) were injected in a 1:1 mixture into mice and the developing tumours were treated with CDDP. Whereas both luciferase activities increased in parallel in the untreated control group, the increase in GLuc activity was strongly diminished by CDDP treatment resulting in a significant drop of the G/C ratio in plasma samples and lysates of explanted tumours ( Fig. 2f–h ). Together these experiments validate GLuc and CLuc as secreted markers that can be measured with high sensitivity and no crosstalk for monitoring competitively the proliferation of two distinct cell populations in mice. 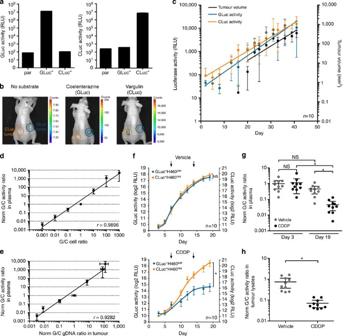Figure 2: Monitoring the dynamics of clonal evolutionin vivowith secreted luciferases. (a) Measurement of GLuc and CLuc in the plasma of mice bearing tumours arising from parental (par), GLuc+or CLuc+HCT116 cells. (b) Bioluminescence images of a single mouse with tumours of GLuc+(right flank) and CLuc+HCT116 cells (left flank) following administration of either coelenterazine (GLuc substrate) or vargulin (CLuc substrate). (c) Mice were subcutaneously injected with 1:1 mixtures of GLuc+and CLuc+HCT116 cells. GLuc and CLuc activity measured in blood plasma and tumour volume measured with calipers are shown. (d,e) Mice were subcutaneously injected with indicated mixtures of GLuc+and CLuc+HCT116 cells (n=10 mice per cell mixture). GLuc/CLuc activity ratio in the plasma of tumour-bearing mice correlates with injected cell ratio (d) and cell ratio determined by GLuc/CLuc-qPCR on genomic DNA isolated from explanted tumours (e). (f–h) Mice were subcutaneously injected with a 1:1 mixture of GLuc+H460parand CLuc+H460rescells and treated with CDDP on day 7 and day 14. (f) GLuc and CLuc activity in the plasma (mean±s.e.m.). Tumour growth curves were analysed by two-way analysis of variance (*P<0.001). (g) GLuc/CLuc activity ratio in plasma (mean±95% confidence interval; *,P<0.01, nonparametric Kruskal–Wallis test and Dunn’s post test for multiple comparisons). (h) GLuc/CLuc activity ratio in tumour lysate (mean±95% confidence interval; *P<0.0001, nonparametric Kolmogorov–Smirnov test). Data are presented as mean±s.d. unless indicated otherwise. Correlation is indicated by the Pearson’s correlation coefficientr. Figure 2: Monitoring the dynamics of clonal evolution in vivo with secreted luciferases. ( a ) Measurement of GLuc and CLuc in the plasma of mice bearing tumours arising from parental (par), GLuc + or CLuc + HCT116 cells. ( b ) Bioluminescence images of a single mouse with tumours of GLuc + (right flank) and CLuc + HCT116 cells (left flank) following administration of either coelenterazine (GLuc substrate) or vargulin (CLuc substrate). ( c ) Mice were subcutaneously injected with 1:1 mixtures of GLuc + and CLuc + HCT116 cells. GLuc and CLuc activity measured in blood plasma and tumour volume measured with calipers are shown. ( d , e ) Mice were subcutaneously injected with indicated mixtures of GLuc + and CLuc + HCT116 cells ( n =10 mice per cell mixture). GLuc/CLuc activity ratio in the plasma of tumour-bearing mice correlates with injected cell ratio ( d ) and cell ratio determined by GLuc/CLuc-qPCR on genomic DNA isolated from explanted tumours ( e ). ( f – h ) Mice were subcutaneously injected with a 1:1 mixture of GLuc + H460 par and CLuc + H460 res cells and treated with CDDP on day 7 and day 14. ( f ) GLuc and CLuc activity in the plasma (mean±s.e.m.). Tumour growth curves were analysed by two-way analysis of variance (* P <0.001). ( g ) GLuc/CLuc activity ratio in plasma (mean±95% confidence interval; *, P <0.01, nonparametric Kruskal–Wallis test and Dunn’s post test for multiple comparisons). ( h ) GLuc/CLuc activity ratio in tumour lysate (mean±95% confidence interval; * P <0.0001, nonparametric Kolmogorov–Smirnov test). Data are presented as mean±s.d. unless indicated otherwise. Correlation is indicated by the Pearson’s correlation coefficient r . Full size image Monitoring shRNA-induced tumour heterogeneity under therapy Tumour relapse after therapy can be caused by resistance-mediating genetic alterations in preexisting or therapy-induced subclones that overgrow the majority of sensitive clones [3] . To explore the impact of a single gene on clonal tumour evolution, we designed lentiviral vectors that genetically couple expression of GLuc or CLuc to the expression of a target-specific shRNA in the miR30 backbone ( Fig. 3a ) [26] . To test the system, we used shRNAs targeting the tumour suppressor p53 as a critical mediator of tumour therapy [27] . GLuc-coupled expression of two independent p53-targeting shRNAs (GLuc + shp53) reduced induction of p53 and its target gene p21/CDKN1A by the MDM2 inhibitor nutlin-3a in p53 wild-type HCT116 cells ( Fig. 3b ). Cells expressing non-targeting control shRNAs (nsh) coupled to either GLuc (GLuc + nsh) or CLuc (CLuc + nsh) served as controls. We mixed GLuc + shp53 or GLuc + nsh cells 1:1 with CLuc + nsh cells as reference. The G/C ratio in the cell culture supernatant of all these mixtures remained stable over 10 days in untreated cells ( Fig. 3c ). In contrast, in GLuc + shp53 mixtures that were exposed to nutlin-3a the G/C ratio increased progressively consistent with resistance of GLuc + shp53 cells ( Fig. 3c ). No change in the G/C ratio was observed in a parallel control experiment with p53-knockout HCT116 cells that fail to respond to nutlin-3a treatment ( Supplementary Fig. 5 ). A ‘flip-color’ design, labelling nsh HCT116 p53 +/+ reference cells with GLuc and shp53 cells with CLuc, yielded the expected inverse result—a progressive decrease in the G/C ratio when cell mixtures were treated with the DNA damaging drug 5-fluorouracil—indicating that both luciferases can be used interchangeably ( Supplementary Fig. 6 ). When 1:1 mixtures of GLuc + shp53 and CLuc + nsh cells were used to generate tumours in mice, both GLuc and CLuc activities increased in vehicle-treated animals with similar kinetics ( Fig. 3d ). Consistent with resistance of GLuc + shp53 cells to nutlin-3a, GLuc—but not CLuc—activity increased progressively in nutlin-3a-treated mice resulting in a significantly elevated G/C plasma ratio in the end ( Fig. 3d,e ). Immunohistochemistry for p53 and GLuc on tumour sections confirmed the enrichment of GLuc + shp53 cells in nutlin-3a-treated tumours relative to the mixture of GLuc + shp53 and p53-positive CLuc + nsh cells in vehicle-treated tumours ( Fig. 3f ). We conclude that coupled expression of shRNAs and secreted luciferases can be used to monitor the effects of a gene on clonal tumour evolution under therapy in both cell culture and mouse models. 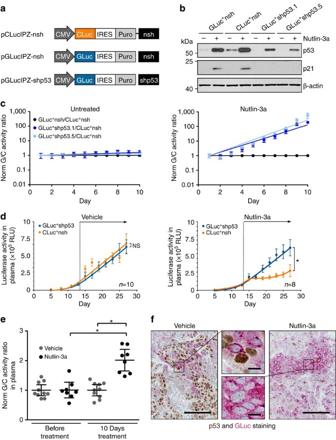Figure 3: Monitoring evolution of shRNA-induced tumour heterogeneity under therapy. (a) Lentiviral vectors for constitutive, coupled expression of shRNAs with GLuc or CLuc. (b) Western blot for p53, p21 (Cdkn1a) and β-actin (control) in HCT116 cells transduced with the indicated shRNA luciferase vectors following treatment with nutlin-3a. (c) GLuc/CLuc activity ratio in the supernatant of the indicated mixed cell cultures in the absence (left) and presence (right) of nutlin-3a. G/C ratios were normalized to the GLuc+nsh/CLuc+nsh control mixture (n=3). (d) Mice were injected subcutaneously with a 1:1 mixture of GLuc+shp53/CLuc+nsh HCT116 cells and treated with vehicle (left) or nutlin-3a (right) starting on day 13. Shown is the mean GLuc and CLuc activity in the plasma (±s.e.m.). Tumour growth curves were analysed by two-way analysis of variance (*P<0.005). (e) GLuc/CLuc plasma ratio (mean±95% confidence interval; *P<0.01, nonparametric Kruskal–Wallis test and Dunn’s post test for multiple comparisons). (f) Immunohistochemistry for p53 (brown) and GLuc (red) in representative tumours explanted from vehicle or nutlin-3a-treated mice. Large scale bars, 100 μm; small scale bars, 10 μm. All data are presented as mean±s.d. unless indicated otherwise. Figure 3: Monitoring evolution of shRNA-induced tumour heterogeneity under therapy. ( a ) Lentiviral vectors for constitutive, coupled expression of shRNAs with GLuc or CLuc. ( b ) Western blot for p53, p21 (Cdkn1a) and β-actin (control) in HCT116 cells transduced with the indicated shRNA luciferase vectors following treatment with nutlin-3a. ( c ) GLuc/CLuc activity ratio in the supernatant of the indicated mixed cell cultures in the absence (left) and presence (right) of nutlin-3a. G/C ratios were normalized to the GLuc + nsh/CLuc + nsh control mixture ( n =3). ( d ) Mice were injected subcutaneously with a 1:1 mixture of GLuc + shp53/CLuc + nsh HCT116 cells and treated with vehicle (left) or nutlin-3a (right) starting on day 13. Shown is the mean GLuc and CLuc activity in the plasma (±s.e.m.). Tumour growth curves were analysed by two-way analysis of variance (* P <0.005). ( e ) GLuc/CLuc plasma ratio (mean±95% confidence interval; * P <0.01, nonparametric Kruskal–Wallis test and Dunn’s post test for multiple comparisons). ( f ) Immunohistochemistry for p53 (brown) and GLuc (red) in representative tumours explanted from vehicle or nutlin-3a-treated mice. Large scale bars, 100 μm; small scale bars, 10 μm. All data are presented as mean±s.d. unless indicated otherwise. Full size image Monitoring clonal evolution during metastasis In contrast to the tumour suppressive activity of wild-type p53, mutant p53 (p53mut) exhibits an oncogenic gain-of-function leading to enhanced metastatic potential of tumour cells [28] . We therefore used the same constructs as before to explore whether the dual-secreted luciferase system can also be used to analyse clonal evolution during metastasis. For this, p53-mutated MDA-MB-231 cells were labelled with GLuc or CLuc in combination with control or p53-targeting shRNAs. GLuc + shp53 or GLuc + nsh cells were mixed with CLuc + nsh reference cells and i.v. injected into mice to model metastatic lung colonization. Consistent with the known role of p53mut in this model [28] , bioluminescence GLuc imaging demonstrated extensive colonization of the lungs by GLuc + nsh cells but poorly by p53mut-depleted (GLuc + shp53) cells ( Fig. 4a ). As in vivo bioimaging of the CLuc + nsh reference cells was precluded by high luciferase signals from the blood and attenuation of the blue light emitted from GLuc + and CLuc + labelled lung metastases ( Supplementary Fig. 7 ), we measured GLuc and CLuc activities also ex vivo in lung lysates and by bioluminescence imaging of explanted lungs ( Fig. 4b–d ). While all three cell mixtures generated comparable CLuc signals, GLuc activity was lower in the lungs containing GLuc + shp53 cells resulting in a significantly reduced G/C ratio. Reduced lung colonization by GLuc + shp53 cells was independently confirmed by immunohistochemistry for p53 and GLuc ( Fig. 4e ). In addition to these endpoint assays, monitoring of GLuc and CLuc activities in the plasma revealed a parallel increase of GLuc and CLuc activity in mixtures of GLuc + nsh and CLuc + nsh cells ( Fig. 4f ). In contrast, mice injected with mixtures containing GLuc + shp53 cells showed a weaker increase in GLuc than CLuc activity ( Fig. 4g,h ). We conclude that the dual-secreted luciferase assay can be used to investigate the effects of a gene on tumour metastasis in both endpoint and time course experiments in vivo . 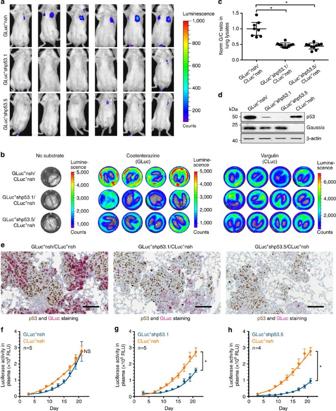Figure 4: Monitoring clonal evolution during metastasis. (a–h) Mice were injected i.v. with the MDA-MB-231 cell mixtures GLuc+nsh/CLuc+nsh, GLuc+shp53.1/CLuc+nsh or GLuc+shp53.5/CLuc+nsh. (a) Bioluminescencein vivoimaging of GLuc activity with coelenterazine. (b) GLuc (coelenterazine) and CLuc (vargulin) imaging of explanted lungs. (c) GLuc/CLuc activity ratios in lung lysates (mean±95% confidence interval; *P<0.01, nonparametric Kruskal–Wallis test and Dunn’s post test for multiple comparisons). (d) Western blot for knockdown efficiency of experimental shRNAs. (e) Immunohistochemical double staining for p53 (brown) and GLuc (red) in lungs explanted from mice injected with (left) GLuc+nsh/CLuc+nsh, (middle) GLuc+shp53.1/CLuc+nsh, and (right) GLuc+shp53.5/CLuc+nsh cell mixtures. Scale bars, 100 μm. (f–h) GLuc/CLuc plasma activity (mean±s.e.m.). Tumour growth curves were analysed by two-way analysis of variance (*P<0.005). Figure 4: Monitoring clonal evolution during metastasis. ( a – h ) Mice were injected i.v. with the MDA-MB-231 cell mixtures GLuc + nsh/CLuc + nsh, GLuc + shp53.1/CLuc + nsh or GLuc + shp53.5/CLuc + nsh. ( a ) Bioluminescence in vivo imaging of GLuc activity with coelenterazine. ( b ) GLuc (coelenterazine) and CLuc (vargulin) imaging of explanted lungs. ( c ) GLuc/CLuc activity ratios in lung lysates (mean±95% confidence interval; * P <0.01, nonparametric Kruskal–Wallis test and Dunn’s post test for multiple comparisons). ( d ) Western blot for knockdown efficiency of experimental shRNAs. ( e ) Immunohistochemical double staining for p53 (brown) and GLuc (red) in lungs explanted from mice injected with (left) GLuc + nsh/CLuc + nsh, (middle) GLuc + shp53.1/CLuc + nsh, and (right) GLuc + shp53.5/CLuc + nsh cell mixtures. Scale bars, 100 μm. ( f – h ) GLuc/CLuc plasma activity (mean±s.e.m.). Tumour growth curves were analysed by two-way analysis of variance (* P <0.005). Full size image Validating essential tumour genes Essential tumour genes are attractive targets for tumour therapy. Knockdown of these genes often compromises tumour cell viability so rapidly that constitutive expression of shRNAs coupled to GLuc/CLuc is prevented. For example, knockdown of cancer proliferation genes like polo-like kinase 1 (PLK1) or Mdm2 results in rapid apoptosis or cell cycle arrest and thus impedes selection and expansion of stable knockdown cells for further analysis [29] . We therefore employed the pINDUCER vector system for dox-regulated shRNA expression and adapted it to the GLuc/CLuc secreted luciferase system ( Fig. 5a ) [30] . HCT116 cells transduced with dox-inducible GLuc- or CLuc-expressing shRNA vectors showed high-level induction of luciferase activities upon dox treatment with negligible background activity in the absence of doxycyclin ( Fig. 5b ). This enabled transduction, selection and expansion of cells with inducible expression of various Mdm2 or PLK1 shRNAs coupled to GLuc. Addition of dox resulted in Mdm2-knockdown followed by p53 stabilization and p21 induction ( Fig. 5c ). PLK1 knockdown resulted in histone H3S10 phosphorylation, indicative of mitotic arrest, and apoptosis ( Fig. 5d , Supplementary Fig. 8 ). In competitive co-cultures of GLuc + shMdm2 or GLuc + shPLK1 with CLuc + nsh cells as reference, the G/C ratio in the supernatant progressively dropped in correlation with knockdown efficiency, indicating depletion of GLuc + shMdm2 and GLuc + PLK1sh cells from the culture ( Fig. 5e,f ). As a proof of specificity, the decrease in the G/C ratio was p53-dependent for Mdm2 but not for PLK1. Furthermore, the PLK1 knockdown could be titrated with increasing dox concentrations, resulting in a dose-dependent decrease in the G/C ratio ( Fig. 5g–i ). 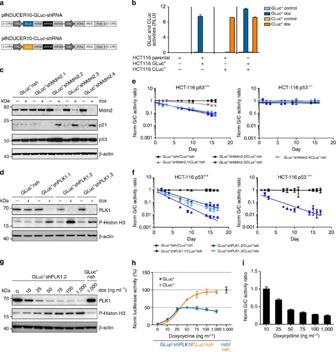Figure 5: Validating essential tumour genes in cell culture. (a) Lentiviral vectors for dox-inducible, coupled expression of shRNAs with GLuc or CLuc. (b) GLuc and CLuc activity measured in the supernatant of uninduced (control) and induced (dox) mixtures of parental, GLuc+and/or CLuc+HCT116 cells. (c,d) Western blot of HCT116 cells transduced with the indicated shRNA-coupled luciferase vectors in the absence and presence of dox. (e,f) GLuc/CLuc activity ratio in the supernatant of the indicated dox-treated mixtures of shRNA+luciferase expressing HCT116 p53+/+(left) and p53−/−(right) cells (n=3). (g) Western blot demonstrating dox titration of PLK1 knockdown. (h) Dox-dependent luciferase activities in supernatant of GLuc+shPLK1/CLuc+nsh cell mixture (n=3). Data were normalized to the dox-induced GLuc+nsh/CLuc+nsh reference mixture set as 100%. (i) Dox-dependency of the GLuc/CLuc activity ratio in the supernatant of the GLuc+shPLK1/CLuc+nsh cell mixture (n=3). All data are presented as mean±s.d. unless indicated otherwise. Figure 5: Validating essential tumour genes in cell culture. ( a ) Lentiviral vectors for dox-inducible, coupled expression of shRNAs with GLuc or CLuc. ( b ) GLuc and CLuc activity measured in the supernatant of uninduced (control) and induced (dox) mixtures of parental, GLuc + and/or CLuc + HCT116 cells. ( c , d ) Western blot of HCT116 cells transduced with the indicated shRNA-coupled luciferase vectors in the absence and presence of dox. ( e , f ) GLuc/CLuc activity ratio in the supernatant of the indicated dox-treated mixtures of shRNA+luciferase expressing HCT116 p53 +/+ (left) and p53 −/− (right) cells ( n =3). ( g ) Western blot demonstrating dox titration of PLK1 knockdown. ( h ) Dox-dependent luciferase activities in supernatant of GLuc + shPLK1/CLuc + nsh cell mixture ( n =3). Data were normalized to the dox-induced GLuc + nsh/CLuc + nsh reference mixture set as 100%. ( i ) Dox-dependency of the GLuc/CLuc activity ratio in the supernatant of the GLuc + shPLK1/CLuc + nsh cell mixture ( n =3). All data are presented as mean±s.d. unless indicated otherwise. Full size image When mixtures of GLuc + shMdm2, GLuc + shPLK1 or GLuc + nsh with CLuc + nsh cells were subcutaneously injected into mice, GLuc and CLuc activities in the plasma remained low until coupled expression of luciferases and shRNAs was induced by dox administration ( Fig. 6a ). Under dox, CLuc activity increased further in all mice. GLuc activity was also induced by dox in all mice initially, indicating that GLuc + cells had expanded and contributed to tumour growth in the absence of dox just as CLuc + cells. While GLuc activity in blood plasma increased even further in mice with GLuc + nsh tumours, it dropped in mice with GLuc + shMdm2 or GLuc + shPLK1 tumours, consistent with a negative selection of Mdm2- or PLK1-knockdown cells during tumour growth in vivo . At the end of the experiment, the tumours were explanted. By measuring luciferase activities in tumour lysates ( Fig. 6b ) and by qPCR-based quantification of GLuc and CLuc copy numbers in tumour DNA ( Fig. 6c ), we confirmed a strongly reduced abundance of the GLuc + MDM2sh and GLuc + PLK1sh tumour subclones relative to the CLuc + nsh reference clone. Importantly, G/C luciferase activity ratios measured in plasma samples correlated well with subclone ratios quantified by qPCR ( Fig. 6d ). We conclude that dox-inducible expression of shRNAs coupled to secreted luciferases provides a sensitive tool to validate a gene as an essential tumour gene in vivo . 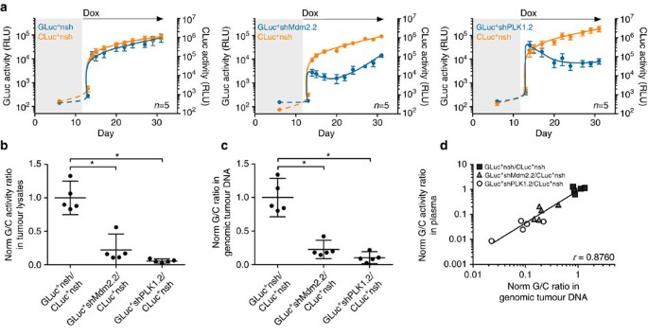Figure 6: Validating essential tumor genesin vivo. (a) Mice were injected subcutaneously with HCT116 cell mixtures (GLuc+nsh/CLuc+nsh, GLuc+shMDM2.2/CLuc+nsh or GLuc+shPLK1.2/CLuc+nsh) and treated with dox starting on day 13. Shown are luciferase activities in blood plasma (mean±s.e.m.). (b) GLuc/CLuc activity ratio in tumour lysates (mean±95% confidence interval; *P<0.01, nonparametric Kolmogorov–Smirnov test). (c) GLuc/CLuc copy number ratio in genomic tumour DNA (mean±95% confidence interval; *P<0.01, nonparametric Kolmogorov–Smirnov test). (d) Correlation of G/C luciferase activity ratio in plasma with G/C copy number ratio in genomic tumor DNA. Correlation is indicated by the Pearson’s correlation coefficientr. Figure 6: Validating essential tumor genes in vivo . ( a ) Mice were injected subcutaneously with HCT116 cell mixtures (GLuc + nsh/CLuc + nsh, GLuc + shMDM2.2/CLuc + nsh or GLuc + shPLK1.2/CLuc + nsh) and treated with dox starting on day 13. Shown are luciferase activities in blood plasma (mean±s.e.m.). ( b ) GLuc/CLuc activity ratio in tumour lysates (mean±95% confidence interval; * P <0.01, nonparametric Kolmogorov–Smirnov test). ( c ) GLuc/CLuc copy number ratio in genomic tumour DNA (mean±95% confidence interval; * P <0.01, nonparametric Kolmogorov–Smirnov test). ( d ) Correlation of G/C luciferase activity ratio in plasma with G/C copy number ratio in genomic tumor DNA. Correlation is indicated by the Pearson’s correlation coefficient r . Full size image Non-invasive monitoring of tumour development in mice usually requires sophisticated imaging techniques for detection of fluorescent or bioluminescent markers [18] . However, quantification of these markers as a measure of tumour mass is hampered by absorption of light in the surrounding tissues. As photon absorption is a function of wavelength, depth and tissue type, quantitative in vivo tracing of cell populations labelled with different markers is therefore, in spite of considerable technical advances, inherently biased [18] , [31] . Furthermore, emission imaging requires expensive instrumentation, is time consuming, involves frequent anaesthesia and repeated systemic substrate injections [18] . Markers that are secreted from tumour cells and measurable in small volumes of blood ex vivo provide considerable advantage. Factors naturally secreted selectively from tumour cells, the so-called ‘tumour markers’, are therefore routinely used in a clinical setting for tumour screening, monitoring of tumour therapy and detection of relapse. It has been reported previously that a secreted luciferase from GLuc can be used as an artificial marker to label tumour cells and monitor tumour growth and therapy response experimentally in small animal models [22] , [23] . Importantly, as GLuc secretion is an active energy-consuming process and the half-life of GLuc in circulation is only approximately 10 min, GLuc activity in the blood is a measure of the total number of viable tumour cells in the organism [22] . Here, we describe and validate the use of GLuc together with CLuc, a second secreted luciferase from Cypridina noctiluca, as a dual reporter system to monitor two distinct cell populations in cell culture and small animals. Competitive tracking of two distinct cell populations reduces the number of required animals by at least 50% and possibly even further as analysing test and control cells in a single animal is expected to reduce experimental variance. In addition, compared with immobilization of animals by anaesthesia for bioimaging, tail vein puncture for blood sampling is less invasive and therefore better suited to monitor processes that require repeated analysis at short time intervals. Furthermore, GLuc and CLuc plasma levels rise earlier than tumours become visible or palpable, allowing tumour therapy studies at less advanced and burdening tumour stages. We therefore believe that the dual reporter system contributes to an improved humane animal experimentation as defined by Russell and Burch [32] . Of note, quantitative measurement of total tumour burden occurs at the expense of bioimaging performance. Tumour localization in the living animal with GLuc and CLuc is limited to near surface detection (such as subcutaneous tumours) or sizeable tumour masses in the interior as the blue light emitted from small tumour nodules in internal organs is attenuated by surrounding tissues and masked by luciferases circulating in the blood stream [33] . The use of secreted variants of red-shifted luciferases is expected to improve bioimaging quality. By expressing GLuc and CLuc together with shRNAs, we can couple cell labelling to genetic manipulation enabling us to interrogate the function of specific genes in tumour development, tumour progression, metastasis and therapy response. By generating genetic heterogeneity, the system is therefore suitable for exploring the dynamic process of clonal tumour evolution as a central cause of phenotypic tumour plasticity and therapy resistance [3] . Plasmids Lentiviral vectors for stable, constitutive expression of GLuc, CLuc and shRNAs were derived from the lentiviral vector pGIPZ (Open Biosystems). To create a unique EcoRI restriction site, the EcoRI site in the pGIPZ plasmid backbone was destroyed. GLuc/CLuc were transferred from pGLuc-Basic (NEB N8082S) and pCLuc-Basic2 (NEB N0317S), respectively, via SbfI/NotI into pPRIME-CMV-dsRed-recipient (Stephen Elledge, Addgene plasmid 11658) generating pPRIME-CMV-GLuc/CLuc. In a second step, CMV-GFP in pGIPZ was substituted by CMV-GLuc/CLuc from pPRIME-CMV-GLuc/CLuc via NotI/XbaI digestion and ligation. The resulting constructs, pGLucIPZ-nsh or pCLucIPZ-nsh, contain sequences for production of lentiviral constructs for stable expression of either GLuc or CLuc and non-silencing control shRNAs, and additionally conferring puromycin resistance to transduced cells. For knockdown of p53, non-silencing shRNAs from pGLucIPZ-nsh or pCLucIPZ-nsh were replaced by p53-targeting shRNAs (shp53.1(V2LHS_217), shp53.5(V3LHS_333920), Open Biosystems) via EcoRI/XhoI restriction sites. To obtain lentiviral vectors for inducible expression of luciferases and shRNAs, the pINDUCER10 vector containing PheS stuffer sequence in the EcoRI/XhoI site [30] was modified: tRFP was replaced by GLuc or CLuc from pCR-Blunt II-TOPO-GLuc or pCR-Blunt II-TOPO-CLuc via restriction digest with AgeI/NotI and ligation. For pCR-Blunt II-TOPO-GLuc or pCR-Blunt II-TOPO-CLuc, luciferases were amplified by PCR (primer sequences 5′-ACCGGTCAAGCTTGGTACC-3′ and 5′-GCATCTTACTTGGCATGACAGTAAG-3′) from pGLuc-Basic (NEB N8082S) and pCLuc-Basic2 (NEB N0317S). For cloning shRNAs, PheS was replaced by shRNAmirs from pGIPZ vectors (Open Biosystems) by EcoRI/XhoI restriction and ligation: shMdm2.1(V2LHS_251529), shMdm2.2(V2LHS_151656), shMdm2.3(V2LHS_379468), shMdm2.4(V2LHS_379469), shPLK1.1(V2LHS_19708), shPLK1.2(V2LHS_19709), shPLK1.3(V2LHS_19711). Lentiviral vector plasmids for constitutive and inducible expression of GLuc or CLuc coupled to shRNAs are available upon request or through Addgene: pCLucIPZ constitutive expression (ID 53222), and pIND-CLucZ tet-inducible expression (ID 53224). Lentiviruses 293T cells were transfected using Arrest-In (Thermo Scientific) with lentiviral vector plasmids and packaging plasmids pMD2.G and psPAX2 (Didier Trono, Addgene plasmids 12259 and 12260). Supernatants containing lentiviruses were collected on the second and third day after transfection and concentrated by polyethylene glycol precipitation [34] . For lentiviral transduction, HCT116, H460 or MDA-MB-231 cells were seeded on six-well plates and infected with concentrated lentivirus in the presence of polybrene (8 μg ml −1 ) and spin infection (1 h, 1,500 r.p.m., 37 °C). Cells were selected with puromycin (1 μg ml −1 ) for 5 days. Cell culture All cell lines were obtained from the American Tissue Collection Center (ATCC) and cultured in high-glucose Dulbecco’s Modified Eagle’s Medium (HCT116, MDA-MB-231) or Roswell Park Memorial Institute medium 1640 medium (H460) supplemented with 10% fetal bovine serum, 100 IU ml −1 penicillin, 100 μg ml −1 streptomycin and 0.25 μg ml −1 amphotericin B (Life Technologies) at 37 °C with 5% CO 2 . Transduced cell lines were maintained in 0.5–2.0 μg ml −1 puromycin after selection was completed. For induction of dox-regulated vectors, cell culture medium was supplemented with 1–2 μg ml −1 doxycycline (Sigma). HCT116 cells were treated with 10 μM nutlin-3a (Merck). CDDP was used at 0.5 μg ml −1 , 5-fluorouracil at 375 μM. Luciferase assays with cell culture media Cell mixtures were seeded in triplicates on 24-well plates. Supernatant was collected every 24 h and replaced with fresh medium. Supernatants were stored in a 96-well plate at −20 °C until the end of the experiment. At the end of the experiment, all supernatants were thawed and shaken on a Thermomixer (Eppendorf) for 5 min at room temperature. After a short centrifugation, supernatants were further diluted 1:10–1:200 for luciferase activity measurements. Coelenterazine (PJK, Germany), the substrate for GLuc, was prepared as a 10 mM stock in acidified ethanol (10 ml EtOH+200 μl 6 M HCl). CLuc substrate vargulin (NEB) was prepared according to the manufacturer’s protocol. 5 μl of each diluted supernatant was measured in triplicates on white polypropylene 96-well plates with V-bottom (Greiner) using the Orion II luminometer (Berthold) with automated substrate injection of either 50 μl coelenterazine solution (stock diluted 1:500 in phosphate-buffered saline (PBS)) or 25 μl vargulin solution (stock diluted 1:500 in Biolux Cypridina Luciferase Assay Buffer (NEB) prediluted 1:5 in PBS). In time course experiments, all collected samples were stored at −20 °C and measured together at the end of the experiment with a single batch of reagents without background correction. GLuc/CLuc ratios were normalized to the start of the experiment and the GLuc + nsh/CLuc + nsh reference mixture. qPCR Genomic DNA was isolated and purified from cell cultures or tumour samples with the QIAamp DNA Blood Mini Kit (Qiagen) according to the manufacturer’s protocol. gDNA (100 ng) was used as template for qPCR. GLuc and CLuc were quantified in a multiplex qPCR reaction on a LightCycler 480 (Roche) with Maxima Probe qPCR Master Mix (Thermo). Primers and probes were used at a final concentration of 300 nM and 250 nM, respectively. Amplification protocol: initial activation of the Hot Start Taq Polymerase for 10 min at 95 °C, followed by 40 cycles of 15 s at 95 °C and 60 s at 60 °C. Primer/probe sequences: GLuc_TaqMan _for 5′-GATCGTCGACATTCCTGAGATT-3′; GLuc_TaqMan_rev 5′-GATCGACCTGTGCGATGAA-3′; GLuc_TaqMan_probe [6FAM]TCCATGGGCTCCAAGTCCTTGAAC[BHQ1]; CLuc_TaqMan_for 5′-AGCTGAACGACTCTGCAATAG-3′; CLuc_ TaqMan_rev 5′-CTTGTGGCACACGTTACATTTC-3′; CLuc_TaqMan_probe [JOE]TCGCCGGTCAAAGTGATCTTGATCA[BHQ1]. Western blots Cells were lysed in NP-40 Lysis Buffer (50 mM Tris-HCl, 150 mM NaCl, 5 mM EDTA, 2% NP-40, pH 8.0) supplemented with protease inhibitor (complete ULTRA tablets EASYpack, Roche) and phosphatase inhibitor (PhosSTOP, Roche). Protein yield was determined by Bradford assay (Biorad). Total protein (30–50 μg) was separated on NuPAGE SDS Gels (Life Technologies) and tank-blotted to nitrocellulose membranes. Following blocking in Tris Buffered Saline with Tween 20 (TBST; 5 mM Tris, 15 mM NaCl, 0.1% Tween 20, pH 7.5) with 10% nonfat dry milk or 5% bovine serum albumin for 1 h, membranes were incubated with primary antibodies diluted in TBST/5% nonfat dry milk or TBST/5% bovine serum albumin and incubated overnight at 4 ° C. Antibodies: α-p53 (SantaCruz DO-1, 1:10,000); α-PLK1 (SantaCruz F-8, sc-17783, 1:200); α-Mdm2 (Hybridoma supernatant (4B2), 1:2); α-p21 (SantaCruz C-19, sc-397, 1:200); α-Phospho-Histone H3 (Ser10) (Cell Signalling #9701, 1:200); α-GLuc (Nanolight 401P, 1:1000); α-actin (Abcam AC-15, 1:5,000). Proteins were detected with secondary antibody (α-mouse IgG-HRP, α-rabbit IgG-HRP from GE Healthcare, 1:3,000) and ECL kit (SuperSignal West Dura Chemiluminescent Substrate, Thermo Scientific). Uncropped scans of representative Western blots are shown in Supplementary Fig. 9 . Animals All animal experiments were performed according to regulations and guidelines of the German Protection of Animals Act and were approved by the Regional Board Giessen. For all xenograft experiments, we used immunocompromised 6–12 week-old Rag2 tm1.1Flv ;Il2rg tm1.1Flv male and female mice kept under SPF conditions. Required sample sizes were calculated by an a priori power analysis. 1 × 10 6 HCT116, MDA-MB-231, or H460 cells were injected subcutaneously or i.v. into the tail vein. For induction of dox-regulated vectors, dox was freshly prepared and given in drinking water in darkened bottles at a concentration of 1 mg ml −1 in H 2 O/2% sucrose. Drinking water was changed every 2nd–3rd day. Nutlin-3a (APAC) was orally administered twice a day at 200 mg kg −1 body weight in 2% Klucel, 0.2% Tween-80 (Fagron). Control mice received 2% Klucel, 0.2% Tween-80 as vehicle control. CDDP was administered intraperitoneally at 7 mg kg −1 body weight in 0.9% NaCl. Luciferase assays with blood plasma 10 μl of blood was obtained by tail vein puncture and mixed directly with 2 μl of 0.125 IE μl −1 heparin. Plasma was collected by centrifugation (15 min, 3,600 g, 4 ° C). For luciferase activity measurements in the Orion II luminometer (Berthold), plasma was diluted 1:10–1:1,000 with PBS. Each diluted sample (5 μl) was measured by injection of 100 μl coelenterazine (stock diluted 1:200 dilution in PBS) or 25 μl vargulin reagent (stock diluted 1:200 in Biolux Cypridina Luciferase Assay Buffer (NEB) prediluted 1:5 in PBS). All plasma samples were measured in duplicates without background correction. In time course experiments, collected plasma samples were stored at −20 °C and measured together at the end of the experiment with a single batch of reagents. Luciferase assays with tumour lysates Tumours were excised from dead mice and minced. Tumour (10–20 mg) was lysed in 100 μl passive lysis buffer (Promega) with the TissueLyser LT (Qiagen). Tumour lysate (5 μl) was measured in duplicate measurements for GLuc and CLuc activity without background correction as described for blood plasma. Bioluminescence imaging Mice were anesthetized with Forane (Baxter). Coelenterazine (50 μg) dissolved in 100 μl PBS was injected i.v. and mice were imaged immediately for 5 min using the IVIS 50 imaging platform (Caliper). Afterwards, mice were i.v. injected with 100 μl of a 1:500 dilution of vargulin (Targeting Systems) and imaged likewise. For ex vivo imaging, lungs were excised, placed in 24-well plates, bathed in 1 ml of coelenterazine reagent (stock diluted 1:1,000 in PBS) and imaged immediately for 1 s. After GLuc imaging, tumours were washed for 1 h in fresh PBS on ice to remove residual coelenterazine. CLuc was detected by adding 1 ml of vargulin solution (stock diluted 1:1,000 in Biolux Cypridina Luciferase Assay Buffer (NEB) prediluted 1:5 in PBS) and imaging for 1 s. Immunohistochemistry Formalin-fixed tumour tissue was embedded in paraffin, cut and fixed on glass slides overnight at 37 °C. Upon antigen retrieval with Tris-EDTA pH 9.0, sections for double staining were blocked in Dual Endogenous Enzyme Blocking Reagent (Dako) and incubated with α-p53 antibody (DO-1, 1:1,000) in Antibody Diluent (Dako REAL) overnight at 4 °C. Biotinylated rabbit-anti-mouse antibody (Dako, E0464, 1:500) served as secondary antibody and was incubated with Streptavidin-labelled Peroxidase (KPL) followed by detection with DAB Plus Reagent Set (Life Technologies). For subsequent GLuc staining, sections were incubated with α-GLuc antibody (Nanolight Technologies 401 P, 1:1,000) at 4 °C overnight. Biotinylated goat-anti-rabbit antibody (Dako, E0432, 1:500) was used as secondary antibody and was detected with Phosphatase-labelled Streptavidin (KPL) and Liquid Permanent Red (Dako). Nuclei were counterstained with Mayersches Haemalaun (Merck) for 15 s before fixation in Mowiol. Statistical analysis All data are presented as mean±s.d. unless indicated otherwise. Correlation is indicated by the Pearson’s correlation coefficient r . Statistical significance of single-time-point experiments was tested using nonparametric tests (Kolmogorov–Smirnov test for two group comparisons; Kruskal–Wallis test and Dunn’s post test for multiple comparisons). Tumour growth curves were analysed by two-way analysis of variance. All statistics were calculated by GraphPad Prism. P <0.05 was considered statistically significant. How to cite this article : Charles, J. P. et al . Monitoring the dynamics of clonal tumour evolution in vivo using secreted luciferases. Nat. Commun. 5:3981 doi: 10.1038/ncomms4981 (2014).